MED18 interaction with distinct transcription factors regulates multiple plant functions Mediator is an evolutionarily conserved transcriptional regulatory complex. Mechanisms of Mediator function are poorly understood. Here we show that Arabidopsis MED18 is a multifunctional protein regulating plant immunity, flowering time and responses to hormones through interactions with distinct transcription factors. MED18 interacts with YIN YANG1 to suppress disease susceptibility genes glutaredoxins GRX480 , GRXS13 and thioredoxin TRX-h5 . Consequently, yy1 and med18 mutants exhibit deregulated expression of these genes and enhanced susceptibility to fungal infection. In addition, MED18 interacts with ABA INSENSITIVE 4 and SUPPRESSOR OF FRIGIDA4 to regulate abscisic acid responses and flowering time, respectively. MED18 associates with the promoter, coding and terminator regions of target genes suggesting its function in transcription initiation, elongation and termination. Notably, RNA polymerase II occupancy and histone H3 lysine tri-methylation of target genes are affected in the med18 mutant, reinforcing MED18 function in different mechanisms of transcriptional control. Overall, MED18 conveys distinct cues to engender transcription underpinning plant responses. Transcriptional control of gene expression underpins many plant processes including responses to the environment. Mediator is an evolutionarily conserved transcriptional cofactor complex in all eukaryotes. Studies in metazoans and yeast suggest that Mediator conveys regulatory information from enhancers and other control elements to the basal RNA polymerase II (RNA Pol II) transcription machinery [1] . Post-translational modifications of specific Mediator subunits can affect global patterns of gene transcription [2] . The plant Mediator, which was first described in 2007, is composed of 21 conserved and 6 plant-specific subunits [3] . As a result, studies on the plant Mediator and its role in plant physiological and cellular functions are in their infancy. MED21, MED8, MED16, MED15 and MED25 are implicated in resistance to necrotrophic pathogens and plant development functions [4] . MED20a, MED18, MED8, and MED17 are implicated in non-coding RNA production [5] . MED18 has been shown to play a role in flowering time and flower organ identity [6] . MED25 has been implicated in diverse functions, including suppression of abscisic acid (ABA) but activation of jasmonic acid (JA) signalling [7] , [8] . MED21 interacts with HUB1 (HISTONE MONOUBIQUITINATION1), an E3 ligase required for ubiquitination of histone H3, modulating plant immune reponses to fungal infection. MED16 is involved in both salicylic acid-mediated systemic acquired resistance and JA/ethylene (JA/ET)-induced pathways affecting responses to Pseudomonas syringae and necrotrophic fungi [9] . MED15 was identified as NON RECOGNITION OF BTH4 and its mutant exhibits insensitivity to salicylic acid but also is impaired in systemic acquired resistance [10] . In these examples, the underlying molecular mechanisms of how Mediator subunits modulate plant functions are not determined. Plant responses to microbial infection is predicated on a timely and coordinated expression of a battery of genes encoding immune response proteins, enzymes and other structural components that restrict pathogen ingress or signal further immune responses. Rapid and extensive perturbations of gene expression follow pathogen infection events and tip the outcome of the interaction to resistance or susceptibility. Thus, transcriptional control is a preeminent component of plant immune response involving transcription factors (TFs), co-activators and permissive or repressive chromatin state [11] . Notably, plant pathogen resistance mechanisms and the transcriptional activation of defence-related genes vary depending on the nature of the pathogen and their virulence mechanisms [12] . Arabidopsis WRKY33, BOS1 (BOTRYTIS SUSCEPTIBLE 1) and RAP2.2 are examples of TFs that promote resistance [13] , [14] , [15] whereas MYB44 and MYB46 suppress resistance to fungal necrotrophs [16] . TFs are also controlled by their co-activators and post-transcriptional regulatory mechanisms. The DNA-binding activity of WRKY33 is controlled by SIB1 (SIGMA FACTOR-BINDING PROTEIN1) and SIB2 (ref. 17) [17] , and its transcription activity is enhanced by MPK3/MPK6 phosphorylation [18] . Modification of histone tails is another layer of transcriptional control that was found to affect plant immune responses [19] , [20] , [21] . Other transcriptional regulators and co-regulators that impact plant immunity have been described in various interactions [11] , [12] . The biological functions of most Mediator subunits remain to be determined. Although it is known in yeast and mammalian cells that MED18 is part of the head module of Mediator, its cellular and physiological functions are not known. Here we demonstrate that Arabidopsis MED18 has a pervasive regulatory impact on multiple plant physiological processes, including plant immunity, flowering time and responses to plant hormones. Underlying the functional versatility of MED18 is its multiple interactions with key and structurally distinct TFs and the recruitment of proteins that regulate transcription. MED18 interacts with zinc finger TF YY1 (YIN YANG1) at the promoters of three plant disease susceptibility genes, glutaredoxins GRXS13 , GRX480 and thioredoxin TRX-h5 , repressing their expression. Accordingly, ectopic expression of one of these, GRX480, results in severe susceptibility to fungal infection. Intriguingly, MED18 is also required for pathogen-induced expression of PTR3, a positive regulator of plant defence. Moreover, MED18 is recruited to ABI5 and FLOWERING LOCUS C ( FLC ) promoters through interaction with TFs ABI4 (ABA INSENSITIVE 4) and SUF4 (SUPPRESSOR OF FRIGIDA4) to regulate responses to ABA and flowering time, respectively. Interestingly, in addition to transcription initiation, MED18 is involved in transcription elongation, termination as well as recruitment of RNA Pol II to target genes in the various pathways. Finally, we demonstrate that MED18 mutation affects the level of H3K36me3 on chromatin of target genes. In sum, we show that MED18 has functions in multiple stages of transcriptional control of gene expression underlying different plant physiological processes. MED18 contributes to plant defence against necrotrophs We screened Arabidopsis Mediator subunits for functions in plant responses to fungal infection. Transfer DNA insertion mutants in Mediator subunits were screened for altered responses to infection by the necrotrophic fungal plant pathogen Botrytis cinerea . In the initial screen, MED18 transfer DNA insertion alleles med18-1 (Sail- 889-C08) and med18-2 (SALK_027178C) were found to be more susceptible to B. cinerea than the wild-type plants ( Fig. 1a,b ). Both lines carry MED18 null alleles with no detectable transcripts ( Supplementary Fig. 1a ). To further ascertain that the observed phenotypes are due to loss of MED18 function, a hemagglutinin (HA)-tagged MED18 construct was transferred into med18-1 mutant ( med18 ; 35S:MED18-HA) and tested for disease resistance. Four days after inoculation (dai) with B. cinerea , med18-1 and med18-2 mutants showed enhanced chlorosis and necrosis, whereas the wild-type plants showed limited disease symptoms ( Fig. 1a ). Expression of MED18-HA restored the disease response phenotype of med18-1 to the wild-type level. At 4 dai, med18-1 and med18-2 accumulated more fungal biomass as measured by the amount of quantitative reverse transcriptase PCR (qRT–PCR) amplification of the constitutive B. cinerea Actin mRNA ( Fig. 1b ). The med18-1;MED18-HA transgenic lines accumulated wild-type level of B. cinerea indicating MED18 enhanced resistance. When inoculated with Alternaria brassicicola , another necrotrophic fungus, the med18 mutant displayed enhanced disease symptoms with significantly larger disease lesions than the wild-type plants ( Fig. 1c,d ). In addition, A. brassisciola grew significantly more in the med18 mutant than in the wild-type plants as measured by the accumulation of the A. brassisciola Cutinase gene (CutA) in qRT–PCR assays ( Fig. 1e ). We conclude that MED18 limits disease symptoms and pathogen growth in plants infected with necrotrophic fungal pathogens. 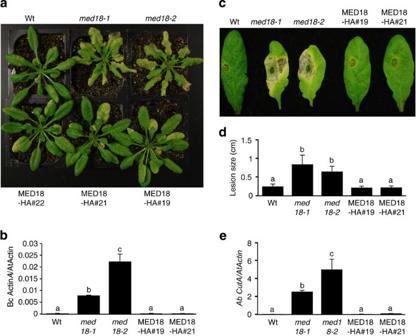Figure 1: MED18 is required for resistance to fungal pathogens. (a)med18mutant exhibits increased disease symptoms, and (b) fungal growth revealing loss of resistance toB. cinerea. (c)med18mutant exhibits increased disease symptoms, (d) size of disease lesion and (e) fungal growth afterA. brassicicolainoculation. Fungal growth was determined by qPCR amplification of theB. cinerea ActinAor theA. brassicicola CutinaseDNA (AbCutA) genes relative to theArabidopsis Actin2gene. The data in (b,e) represent mean values±s.e. from three technical replicates. The quantitative disease data in (d) are mean±s.e. from at least 20 disease lesions. The mean values followed by different letters are significantly different from each other (P<0.01, Student’st-test). The experiments were repeated at least three times with similar results. MED18-HA#19 and #21 are two independent transgenic lines generated in themed18-2mutant background. Wt, wild-type. Figure 1: MED18 is required for resistance to fungal pathogens. ( a ) med18 mutant exhibits increased disease symptoms, and ( b ) fungal growth revealing loss of resistance to B. cinerea . ( c ) med18 mutant exhibits increased disease symptoms, ( d ) size of disease lesion and ( e ) fungal growth after A. brassicicola inoculation. Fungal growth was determined by qPCR amplification of the B. cinerea ActinA or the A. brassicicola Cutinase DNA (Ab CutA ) genes relative to the Arabidopsis Actin2 gene. The data in ( b , e ) represent mean values±s.e. from three technical replicates. The quantitative disease data in ( d ) are mean±s.e. from at least 20 disease lesions. The mean values followed by different letters are significantly different from each other ( P <0.01, Student’s t -test). The experiments were repeated at least three times with similar results. MED18-HA#19 and #21 are two independent transgenic lines generated in the med18-2 mutant background. Wt, wild-type. Full size image The med18 mutant plants displayed no altered responses to the bacterial pathogen P. syringae virulent Pst DC3000 and the nonpathogenic Pst DC3000 hrcC strain, which is defective in type three secretion system ( Supplementary Fig. 2 ). We examined whether MED18 acts within known immune response pathways that mediate responses to necrotrophic fungi. The expression of PDF1.2 gene, a marker for JA/ET-mediated defence responses was enhanced in the med18 mutant relative to the wild-type plants in response to B. cinerea infection or methyl-JA treatment ( Supplementary Fig. 3a,b ). The data indicate that MED18 functions independently of JA signalling or may suppress some responses leading to PDF1.2 gene expression. This is unlike MED25 and MED8 subunits that regulate plant defence through JA signalling [7] , [22] . Thus, MED18 immune response function is mechanistically distinct from previously described Mediator subunits or other defence regulators. MED18 interacts with YY1 to regulate plant immunity To dissect the functions of MED18, we screened for MED18-interacting proteins by yeast-two hybrid assays but no real interactors were identified. Then, we tested MED18 interaction with diverse TFs based on the existing information on gene function. The yeast ( Schizosaccharomyces pombe) MED18 and MED8 have overlapping functions and also form a complex as part of the head module [23] , and MED8 interacts with the zinc finger TFs ACE2p [24] . Because of the overall conservation of Mediator in different eukaryotes, we reasoned that ACE2p orthologs in Arabidopsis may interact with the head module and share the functions of MED18 and MED8. The Arabidopsis YY1 (At4g06634) protein, which was not studied for any biological function in plants, was identified as the best match for the yeast ACE2p. To determine whether Arabidopsis YY1 interacts with MED18 or MED8, we performed a Bimolecular Fluorescence Complementation (BiFC) assay. MED18 and MED8 were each fused to the C-terminal domain of the yellow fluorescent protein (YFP) protein individually (MED18-Yc and MED8-Yc) and YY1 was fused with the N-terminal domain of YFP (YY1-Yn). When MED18-Yc and YY1-Yn were co-expressed in Nicotiana benthamiana leaves, a strong YFP signal was observed in the nucleus as revealed by the co-localization with the nuclear stain 4',6-diamidino-2-phenylindole (DAPI) ( Fig. 2a ). No YFP signal was detected in the control experiment where MED18-Yc was co-expressed with N-YFP alone or when MED8-Yc and YY1-Yn were co-expressed ( Fig. 2a ; Supplementary Fig. 4 ). The interaction between MED18 and YY1 was further verified through co-immunoprecipitation (co-IP) experiments from N. benthamiana plants that transiently co-expressed YY1-HA and Myc-MED18 ( Supplementary Fig 5a ). Co-IP using HA-conjugated beads followed by anti-Myc immuno blot clearly revealed that Myc-MED18 specifically precipitated with YY1-HA. The control experiment where YY1-HA was co-expressed with an empty vector expressing the Myc epitope alone did not show any interaction. 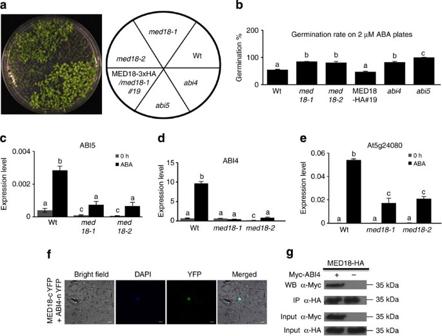Figure 5: MED18 regulates ABA responses through interaction with ABI4. (a)med18mutant plants are insensitive to growth and (b) germination inhibition by ABA. (c) Expression ofABI5, (d)ABI4and (e)At5g24080genes is MED18-dependent. (f) Interaction between MED18-Yc and ABI4-Yn in BiFC assay. (g) Co-immunopreciptation of MED18-HA and Myc-ABI4. MED18-HA was co-expressed with Myc-ABI4 or empty vector containing Myc tag inN. benthamianaleaf as described in the Methods section. In (a)abi4andabi5mutants are included as positive controls. ABA assays were done on MS medium containing 2 μM ABA. The mean values followed by different letters are significantly different from each other (P<0.01, Student’st-test). The experiments were repeated at least three times with similar results. Data represent mean±s.e. (n=3). Scale bars, 10 μm. 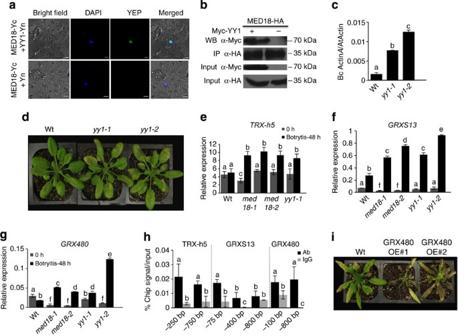In addition, MED18-HA co-precipitated with Myc-YY1 in transgenic Arabidopsis plants expressing both proteins ( Fig. Figure 2: YY1 interacts with MED18 to suppress glutaredoxin and thioredoxin gene expression. (a) BiFC assay showing the interaction between MED18 and YY1. Cells were examined under brightfield (left column), fluorescence (YFP) and as a merged image (right) showing either no interaction or interaction in the nucleus. The nucleus was stained with DAPI (4',6-diamidino-2-phenylindole). (b) Co-IP of MYC-YY1 and MED18-HA. Co-IP experiments were conducted using protein extracts from transgenic plants stably expressing Myc-YY1 and MED18-HA. (c) TheArabidopsis yy1mutant plants support increased fungal growth and (d) disease symptom after inoculation withB. cinerea. (e)TRX-h5,(f)GRXS13and (g)GRX480gene expression in wild-type,med18andyy1mutants. (h) Direct association of YY1 with TRX-h5, GRXS13 and GRX480 promoters revealed by ChIP-qPCR. (i) Increased susceptibility of GRX480 overexpression plants toB. cinerea.The ChIP for Myc-YY1 and chromatin complex was conducted with anti-Myc polyclonal antibody. The disease pictures in (i) are at 6 dai. Gene expression was determined by qPCR using theArabidopsis Actin2gene as a reference for normalization as described51. The mean values followed by different letters are significantly different from each other (P<0.01, Student’st-test). The experiments were repeated at least three times with similar results. Error bars indicate s.e. (n=3). Scale bars, 10 μm. 2b ) Figure 2: YY1 interacts with MED18 to suppress glutaredoxin and thioredoxin gene expression. ( a ) BiFC assay showing the interaction between MED18 and YY1. Cells were examined under brightfield (left column), fluorescence (YFP) and as a merged image (right) showing either no interaction or interaction in the nucleus. The nucleus was stained with DAPI (4',6-diamidino-2-phenylindole). ( b ) Co-IP of MYC-YY1 and MED18-HA. Co-IP experiments were conducted using protein extracts from transgenic plants stably expressing Myc-YY1 and MED18-HA. ( c ) The Arabidopsis yy1 mutant plants support increased fungal growth and ( d ) disease symptom after inoculation with B. cinerea . ( e ) TRX-h5, ( f ) GRXS13 and ( g ) GRX480 gene expression in wild-type, med18 and yy1 mutants. ( h ) Direct association of YY1 with TRX-h5, GRXS13 and GRX480 promoters revealed by ChIP-qPCR. ( i ) Increased susceptibility of GRX480 overexpression plants to B. cinerea. The ChIP for Myc-YY1 and chromatin complex was conducted with anti-Myc polyclonal antibody. The disease pictures in ( i ) are at 6 dai. Gene expression was determined by qPCR using the Arabidopsis Actin2 gene as a reference for normalization as described [51] . The mean values followed by different letters are significantly different from each other ( P <0.01, Student’s t -test). The experiments were repeated at least three times with similar results. Error bars indicate s.e. ( n =3). Scale bars, 10 μm. Full size image Next, we tested the biological function of YY1 with loss-of-function alleles yy1-1 (SALK_071311C) and yy1-2 (SALK_040806C) that produced no YY1 gene transcripts ( Supplementary Fig. 1b ). Four dai, yy1 mutants supported significantly more B. cinerea growth and exhibited enhanced disease symptoms than the wild-type ( Fig. 2c,d ). The disease susceptibility of the yy1 mutant was rescued by YY1-HA expressed from a constitutive promoter revealing that the epitope-tagged protein and constitutive expression of the gene do not affect its functions ( Supplementary Fig. 5b ). Thus, YY1 positively regulates plant defence against B. cinerea, and its function in plant immunity involves interaction with MED18. MED18 interacts with putative repression domain of YY1 The overall domain structure of the Arabidopsis YY1 protein and sequence comparisons are presented in Supplementary Fig. 6 . Arabidopsis YY1 protein contains N-terminus DNA-binding C 2 H 2 -type zinc finger (80–190 aa) and C-terminus SFP1 motifs (210–275 aa) that may function as a transcriptional repressor [25] ( Supplementary Fig. 6a ). To determine the specific region in YY1 protein that is required for its interaction with MED18, the N-terminus of YY1 including the zinc finger motif (1–200 aa) or the SFP1 motif (201–290 aa) were fused to the N-terminal domain of YFP protein (YY1-Zn-Yn, YY1-SFP1-Yn), respectively. BiFC assays show that YY1-SFP1-Yn but not the YY1-Zn-Yn interacts with MED18-Yc ( Supplementary Fig. 6b ). The data suggest that MED18 does not affect the DNA-binding activity of YY1, but may regulate its transcriptional repression function through direct physical interaction. The Arabidopsis YY1 shared significant sequence identity and similarity to metazoan YY1 TFs, particularly in the conserved zinc finger and SFP1 domains ( Supplementary Fig. 6c ). However, no report presents any functional and molecular link between Mediator and the metazoan YY1 proteins. YY1 regulates plant disease susceptibility genes We explored the RNA-seq data (described below) to identify YY1 and MED18 target genes. The expression of Arabidopsis thioredoxin ( TRX-h5, LIV1, LOCUS OF INSENSITIVITY TO VICTORIN) and glutaredoxin (GRXS13, GRX480) genes was closely examined due to their increased expression in the med18 mutant based on RNA-seq data. At 2 dai with B. cinerea , expressions of TRX-h5 , GRXS13 and GRX480 genes were significantly elevated by several fold in both med18 and yy1 mutants ( Fig. 2e–g ). These data are consistent with the repressive functions of YY1 (ref. 25) [25] and suggest that YY1 interactions with MED18 have a repressive outcome. Notably, other stress-related genes show normal expression in the mutant lines. For example, the MPK6 gene that is known to be induced by biotic and abiotic stresses was induced by B. cinerea independent of MED18 and YY1 ( Supplementary Fig. 7 ). The direct transcriptional regulation of GRX and TRX genes by YY1 was further corroborated by chromatin immunoprecipitation (ChIP) experiments in 35S:Myc-YY1 transgenic plants ( Fig. 2h ). The −800 bp and the −100 bp regions of GRX480 promoter, upstream of the transcription start site, was significantly enriched for Myc-YY1 ( Fig. 2h ). Similarly, the −250 bp and −750 bp region in the TRX-h5 promoter and the −75 bp region in GRXS13 promoter were significantly enriched for Myc-YY1. Furthermore, the −400 bp region of the GRXS13 promoter showed moderate enrichment for Myc-YY1. The data demonstrate the direct association of Myc-YY1 with TRX and GRX genes. To test whether enhanced GRX gene expression enhances plant susceptibility to B. cinerea , Arabidopsis transgenic plants which overexpress GRX480 were challenged with B. cinerea . At 6 dai, the GRX480 transgenic plants were completely macerated, but wild type plants remained relatively green ( Fig. 2i ). This data confirmed that elevated expression of GRX and TRX genes contribute to the enhanced susceptibility of the med18 and yy1 mutants to fungal infection. Arabidopsis grxs13 mutant exhibits enhanced resistance to B. cinerea [26] , whereas the trx-h5 mutant is insensitive to the victorin toxin produced by the necrotrophic fungus Cochliobolus victoriae [27] . Interestingly, TRX-h5 is a direct virulence target for the victorin toxin [28] . Elevated expressions of TRX and GRX genes in med18 and yy1 mutants are consistent with their enhanced susceptibility to necrotrophic fungi. GRX and TRX modify the redox status of various target proteins by reducing their disulphide bridges thereby altering their structure and activity [29] . Thus, we conclude that MED18 interacts with YY1 and positively regulates the function of YY1 to suppress the transcription of negative regulators of defence GRXs and TRXs during plant defence against B. cinerea . Impact of MED18 on genome wide gene expression We conducted RNA-seq analysis to understand the extent of the regulatory impact of MED18 and determine whether the phenotypes observed in the med18 mutant were correlated with specific defects in gene expression. RNA- seq data from mock or B. cinerea- inoculated plants were compared as described in the Methods section. Reads per kilobase of exon model per million mapped reads (RPKM) values were calculated for each sample with count data. Then, we adopted a cutoff level of at least twofold change in gene expression and FDR value ( P ≤0.05) to identify Botrytis -induced genes (BIGs) and Botrytis -suppressed genes (BSGs) ( Fig. 3a ). On the basis of this level of stringency, 2,983 B. cinerea- induced and 3,514-suppressed genes were identified in wild-type plants. In the med18 mutant, 4,963 genes were induced and 6,628 genes suppressed by B. cinerea, out of which 2,568 BIGs and 3,231 BSGs are common to both genotypes. Five genes were induced in the wild type but suppressed in med18-2 , and 8 genes are induced in med18-2 but suppressed in wild type in response to B. cinerea . Overall, as presented in the heat map ( Supplementary Fig. 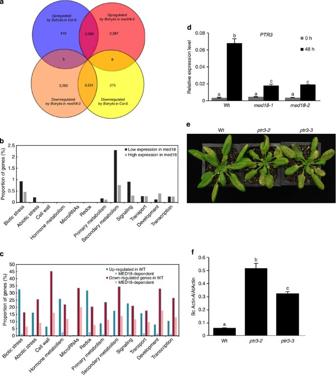8 ), B. cinerea caused significant transcriptional changes in wild-type and med18 mutant plants, but MED18 regulates only a subset of genes because most genes remain at the wild-type level in the infected med18 mutant. Figure 3: RNA-seq analysis determines the global impact and specific targets of MED18 modulating the plant immunity. (a) Venn diagram showing DE of genes in wild-type andmed18mutant plants before and after inoculation withB. cinerea.(b) Proportion of genes in selected functional categories that show increased or decreased basal gene expression in themed18mutant. (c) Proportion of genes in selected functional categories that show MED18-dependent upregulation or downregulation of gene expression in response toB. cinerea.(d) qRT–PCR showing expression ofPTR3duringB. cinereainfection in wild-type andmed18mutant plants. Means followed by different letters are significantly different from each other (P<0.01, Student’st-test). The experiments were repeated at least three times. Error bars indicate s.e. (n=3). (e) Theptr3mutants exhibit enhanced susceptibility and (f) enhanced fungal growth after inoculation withB. cinerea. B. cinereagrowth was determined by qPCR amplification of theB. cinereaActin A (Bc ActinA). The experiments were repeated three times. The data represent mean values±s.e. from three technical replicates. Venn diagram in (a) shows gene responding transcriptionally toB. cinereainfection in MED18-dependent or -independent manner based on analysis of the RNA-seq data. Increase or decrease in transcript abundance was determined based on at least twofold change (P≤0.05,t-test) in inoculated and non-inoculated samples. Ovals represent the number of genes for which transcript levels were changed in response toB. cinerea. The overlap between the ovals shows the number of genes regulated in genotypes and infection-dependent manner. Statistically significant changes were determined by R-package V3.16.5 (P<0.05,t-test). Gene expression was determined by quantitative RT–PCR (qPCR) using theArabidopsis Actin2gene as a reference for normalization as described51. Figure 3: RNA-seq analysis determines the global impact and specific targets of MED18 modulating the plant immunity. ( a ) Venn diagram showing DE of genes in wild-type and med18 mutant plants before and after inoculation with B. cinerea. ( b ) Proportion of genes in selected functional categories that show increased or decreased basal gene expression in the med18 mutant. ( c ) Proportion of genes in selected functional categories that show MED18-dependent upregulation or downregulation of gene expression in response to B. cinerea. ( d ) qRT–PCR showing expression of PTR3 during B. cinerea infection in wild-type and med18 mutant plants. Means followed by different letters are significantly different from each other ( P <0.01, Student’s t -test). The experiments were repeated at least three times. Error bars indicate s.e. ( n =3). ( e ) The ptr3 mutants exhibit enhanced susceptibility and ( f ) enhanced fungal growth after inoculation with B. cinerea. B. cinerea growth was determined by qPCR amplification of the B. cinerea Actin A (Bc ActinA). The experiments were repeated three times. The data represent mean values±s.e. from three technical replicates. Venn diagram in ( a ) shows gene responding transcriptionally to B. cinerea infection in MED18-dependent or -independent manner based on analysis of the RNA-seq data. Increase or decrease in transcript abundance was determined based on at least twofold change ( P ≤0.05, t -test) in inoculated and non-inoculated samples. Ovals represent the number of genes for which transcript levels were changed in response to B. cinerea . The overlap between the ovals shows the number of genes regulated in genotypes and infection-dependent manner. Statistically significant changes were determined by R-package V3.16.5 ( P <0.05, t -test). Gene expression was determined by quantitative RT–PCR (qPCR) using the Arabidopsis Actin2 gene as a reference for normalization as described [51] . Full size image The differentially expressed genes based on fold changes (FDR ≤0.05) were categorized into functional groups based on Gene Ontology. Among these, 12 functional categories were examined in detail for the basal and B. cinerea and/or MED18-dependent expression. The proportion of differentially expressed genes for each category relative to the total number of Arabidopsis genes assigned to that functional category is shown ( Fig. 3b,c ). The proportions of MED18-dependent BSGs in all functional groups tested were consistently higher than those MED18-dependent BIGs. This suggests that MED18 has a greater repressive impact on gene expression after infection by B. cinerea . PTR3 is regulated by MED18 and contributes to defence The expression of 33 genes was at least twofold lower ( P ≤0.05) in B. cinerea- inoculated med18 than in B. cinerea- inoculated wild-type plants based on differential gene expression using RPKM, EdgeR and Voom analysis ( Supplementary Data 1 ). One of these is the PTR3 gene encoding a di- and tri-peptide transporter previously implicated in plant defence against wounding and infection by necrotrophic bacterial pathogens [30] . Analysis of qRT–PCR data confirmed that the PTR3 gene expression in the med18 mutant was significantly lower than that in B. cinerea- inoculated wild-type plants ( Fig. 3d ) suggesting that it is a bona fide MED18 target. To determine whether PTR3 is required for defence against B. cinerea , two transfer DNA insertion alleles ptr3-2 and ptr3-3 were tested for their immune responses. Both PTR3 mutations caused loss-of-function alleles with no wild-type transcripts produced ( Supplementary Fig. 1c ). Four dai, ptr3-2 and ptr3-3 were more susceptible to B. cinerea and the fungus grew significantly more than in the wild-type plants suggesting that PTR3 and MED18 share functions in plant immunity ( Fig. 3e,f ). ChIP-qRT–PCR (ChIP-qPCR) experiments reveal that the regions covering the −500 bp PTR3 promoter, the TATA box, which is the RNA Pol II-binding site, were significantly enriched with MED18-HA ( Fig. 4a ). In the −500 bp region, the mock and B. cinerea- induced samples contained comparable levels of MED18-HA, whereas the TATA box was significantly enriched following B. cinerea inoculation. MED18-HA did not associate with the Arabidopsis Actin2 gene which is expressed constitutively confirming specific association of MED18 with target gene regulatory regions ( Supplementary Fig. 9a ). The data are consistent with the enhanced transcription of PTR3 after B. cinerea infection and that MED18 directly associates with the PTR3 promoter to positively regulate its gene expression. Thus, one of the functions of MED18 in defence is through direct regulation of PTR3 gene expression. 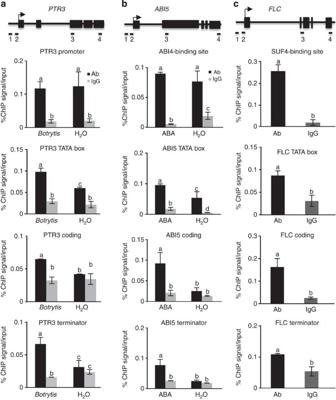Together with the data in the previous section, at least two kinds of mechanisms (impaired PTR3 and elevated TRX and GRX gene expressions) contribute to the disease susceptibility phenotype of med18 mutants. Figure 4: Direct association of MED18 with different regions of target genes. MED18 is recruited to the (a) PTR3, (b) ABI5 and (c) FLC promoter, TATA box, coding and terminator regions. Four 4-week-old plants 2 dai (PTR3), 2-week-old seedlings after ABA treatment (ABI5) or 2-week-old seedlings with no treatment (FLC) were used for isolating input chromatin. ChIP data are from35S:MED18-HA;med18-1transgenic plants. Epitope-tagged MED18-chromatin complex was immunoprecipitated with anti-HA antibody. A control reaction was processed in parallel with mouse IgG. ChIP- and input-DNA samples were quantified by real-time qPCR using primers specific to the different regions of thePTR3,ABI5andFLCgenes. The structures ofPTR3,ABI5andFLCgenes as well as the positions of the primers used for qRT–PCR corresponding to the distal promoter (1), TATA box (2), coding (3) and terminator (4) regions are marked on the diagram at the top. The ChIP results are presented as percentage of input DNA. Error bars indicate s.e. (n=3). The experiments were repeated at least two times with similar results. Figure 4: Direct association of MED18 with different regions of target genes. MED18 is recruited to the ( a ) PTR3, ( b ) ABI5 and ( c ) FLC promoter, TATA box, coding and terminator regions. Four 4-week-old plants 2 dai (PTR3), 2-week-old seedlings after ABA treatment (ABI5) or 2-week-old seedlings with no treatment (FLC) were used for isolating input chromatin. ChIP data are from 35S:MED18-HA;med18-1 transgenic plants. Epitope-tagged MED18-chromatin complex was immunoprecipitated with anti-HA antibody. A control reaction was processed in parallel with mouse IgG. ChIP- and input-DNA samples were quantified by real-time qPCR using primers specific to the different regions of the PTR3 , ABI5 and FLC genes. The structures of PTR3 , ABI5 and FLC genes as well as the positions of the primers used for qRT–PCR corresponding to the distal promoter (1), TATA box (2), coding (3) and terminator (4) regions are marked on the diagram at the top. The ChIP results are presented as percentage of input DNA. Error bars indicate s.e. ( n =3). The experiments were repeated at least two times with similar results. Full size image MED18 regulates responses to plant hormones To gain insight into the specificity and molecular bases of plant defence functions of MED18, we tested the sensitivity of med18 mutant seedlings to various plant hormones. The med18 mutants were insensitive to germination and early growth inhibition by ABA ( Fig. 5a ). Ten days after germination, similar to the well-known ABA insensitive mutants abi4 and abi5, the growth of med18 mutants was not inhibited by ABA. At four days after germination on ABA, more than 80% of med18 mutant seeds germinated whereas only 50% of wild-type seeds germinated ( Fig. 5b ). MED18-HA suppressed the ABA insensitivity of the med18-1 mutant. In the triple response assay where seedlings were grown in the presence of ethylene precursor 1-aminocyclopropane-1-carboxylic acid (ACC), the wild-type seedlings, as expected, displayed exaggerated apical hooks, swollen hypocotyls and inhibition of root and hypocotyl elongation. The med18 mutant lacked the apical hook but displayed the two other features of the triple response ( Supplementary Fig. 10a ). The data indicate that the MED18 mutation partially blocks the plant growth response to ethylene similar to the previously described hookless mutant [31] . Figure 5: MED18 regulates ABA responses through interaction with ABI4. ( a ) med18 mutant plants are insensitive to growth and ( b ) germination inhibition by ABA. ( c ) Expression of ABI5 , ( d ) ABI4 and ( e ) At5g24080 genes is MED18-dependent. ( f ) Interaction between MED18-Yc and ABI4-Yn in BiFC assay. ( g ) Co-immunopreciptation of MED18-HA and Myc-ABI4. MED18-HA was co-expressed with Myc-ABI4 or empty vector containing Myc tag in N. benthamiana leaf as described in the Methods section. In ( a ) abi4 and abi5 mutants are included as positive controls. ABA assays were done on MS medium containing 2 μM ABA. The mean values followed by different letters are significantly different from each other ( P <0.01, Student’s t -test). The experiments were repeated at least three times with similar results. Data represent mean±s.e. ( n =3). Scale bars, 10 μm. Full size image ABI4 recruits MED18 to the ABI5 promoter To understand the molecular mechanisms underlying the altered ABA responses of med18 , we examined the expression of ABI4 and ABI5, regulatory genes in the ABA pathway. The expression of both ABI4 and ABI5 were dramatically lower in med18 mutants than in wild type plants with or without ABA ( Fig. 5c,d ). The data indicate that ABI5 and ABI4 are regulated by MED18, and that the low ABI4 and ABI5 gene expression in med18 mutants may account for its altered ABA responses. In addition, the expression of Arabidopsis At5g24080 gene encoding a serine threonine kinase was significantly reduced in the med18 mutant indicating that MED18 regulates additional genes in the ABA response pathways that may be independent of ABI5 ( Fig. 5e ). The At5g24080 gene expression is completely dependent on ABI4 although its function is unknown [32] . To determine whether MED18 directly regulates the transcription of ABI5 , we tested the recruitment of MED18 to the ABI5 promoter. ChIP-qPCR experiments on med18 ; 35S:MED18-HA transgenic plants reveal that MED18-HA was recruited to the ABI4-binding site on the ABI5 promoter with or without ABA treatment, whereas MED18 recruitment to the TATA box region of ABI5 was significantly enhanced by ABA ( Fig. 4b ). The data indicate that MED18 directly regulates ABI5 gene transcription, and the recruitment of MED18 to the promoter is functionally related to ABI4 and RNA Pol II. ABI4 is known to bind to the ABI5 promoter and enhance its expression [33] . This information prompted us to test whether MED18 directly interacts with ABI4 to regulate ABI5 gene expression. BiFC assays demonstrate the interaction of MED18-Yc and ABI4-Yn as revealed by the YFP signal in the nucleus ( Fig. 5f ). YFP signal was not detected in the control experiment in which MED18-Yc was co-expressed with unfused N-YFP ( Supplementary Fig. 4 ). In addition, MED18 and ABI4 co-IP experiments were performed from N. benthamiana leaves co-expressing Myc-ABI4 and MED18-HA. Co-IP with HA-conjugated beads followed by anti-Myc immune blot indicates that Myc-ABI4 specifically precipitated with MED18-HA but not with the empty vector expressing the Myc epitope alone, and thus confirming the MED18–ABI4 interactions ( Fig. 5g ). We investigated whether the defence and ABA functions of MED18 were linked. The abi5 mutant was clearly more resistant to B. cinerea and abi4 is comparable to wild type ( Supplementary Fig. 10b ) despite their reduced expression in med18. Thus, we conclude that the ABA insensitivity and immune response defects of the med18 mutant are due to independent functions. MED18 regulates flowering through interaction with SUF4 The med18 mutants exhibit delayed flowering under long day (12: 12 h dark: light cycle) and short day conditions (6 h light: 18 h dark cycles) ( Fig. 6a,b ; Supplementary Fig. 11 ). Under long day, med18 mutants flower at about 68 days after germination, compared with wild-type plants that flower at 45 days ( Fig. 6b ). The late flowering was also clearly manifested in leaf number; med18 mutants produced about 96 rosette leaves at flowering compared with the wild-type plants that produced only about 35 leaves ( Fig. 6c ). The late-flowering phenotypes of the med18 mutant were recently described [6] . To explore the molecular basis of the late-flowering phenotype of med18 mutant, we tested the expression level of important flowering genes FLC , a negative regulator of flowering, and FT ( FLOWERING LOCUS T ) and SOC1 ( SUPPRESSOR OF OVEREXPRESSION OF CO1 ), two genes promoting flowering ( Fig. 6d ). Analysis of qRT–PCR data indicated that FT and SOC are expressed at a lower level in the med18 mutant than in the wild type. FLC expression was dramatically higher in med18 mutants than in wild-type plants ( Fig. 6d ). The late flowering phenotype could thus be attributed to the elevated FLC but the suppressed expression of SOC and FT by FLC. 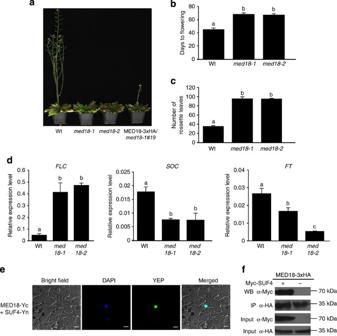Figure 6: MED18 modulates flowering time through interaction with SUF4 and by regulating FLC. (a) Delayed flowering inmed18mutant relative to the wild-type plants. (b) Days to flowering and (c) number of rosette leaves revealing delayed flowering of themed18. (d) Expression ofFLC, SOCandFTgenes in wild type andmed18.(e) BiFC assay showing interaction between MED18 and SUF4. (f) Co-IP of Myc-SUF4 and MED18-HA. Co-IP experiments were conducted using transgenic plants stably expressing Myc-SUF4 and MED18-HA. The co-IP experiments and the qRT–PCR were performed as described in the legend forFig. 2and in the Methods section. Leaf numbers were counted at bolting. The significance of the differences between mean values for the days to flowering, qRT–PCR data and number of rosette leaves was tested (P<0.01, Student’st-test). All experiments were repeated at least three times with similar results. Scale bars, 10 μm. The rosette leaf number (b) and days to flowering (c) data for wild type andmed18mutants are from at least 60 plants. The gene expression data (d) were determined by quantitative qPCR using theArabidopsis Actin2gene as a reference for normalization. The mean values followed by different letters are significantly different from each other (P<0.01, Student’st-test). Error bars indicate s.e. (n=3). Figure 6: MED18 modulates flowering time through interaction with SUF4 and by regulating FLC. ( a ) Delayed flowering in med18 mutant relative to the wild-type plants. ( b ) Days to flowering and ( c ) number of rosette leaves revealing delayed flowering of the med18 . ( d ) Expression of FLC, SOC and FT genes in wild type and med18. ( e ) BiFC assay showing interaction between MED18 and SUF4. ( f ) Co-IP of Myc-SUF4 and MED18-HA. Co-IP experiments were conducted using transgenic plants stably expressing Myc-SUF4 and MED18-HA. The co-IP experiments and the qRT–PCR were performed as described in the legend for Fig. 2 and in the Methods section. Leaf numbers were counted at bolting. The significance of the differences between mean values for the days to flowering, qRT–PCR data and number of rosette leaves was tested ( P <0.01, Student’s t -test). All experiments were repeated at least three times with similar results. Scale bars, 10 μm. The rosette leaf number ( b ) and days to flowering ( c ) data for wild type and med18 mutants are from at least 60 plants. The gene expression data ( d ) were determined by quantitative qPCR using the Arabidopsis Actin2 gene as a reference for normalization. The mean values followed by different letters are significantly different from each other ( P <0.01, Student’s t -test). Error bars indicate s.e. ( n =3). Full size image FLC gene expression is regulated through multiple mechanisms, and its increased expression may be a consequence of direct or indirect regulation by MED18. To resolve this, the recruitment of MED18 to the FLC promoter was examined by ChIP-qPCR as described in the previous sections. We tested the association of MED18-HA with the region covering the TATA box as well as the −500 bp region which is the binding site of SUF4, a TF positively regulating FLC gene expression [34] . MED18 was recruited not only to the TATA box but also to the SUF4-binding site of the FLC promoter ( Fig. 4c ) indicating that FLC is a direct target of MED18. This observation also suggested a possible interaction between MED18 and SUF4, analogous to the YY1-MED18 and ABI4-MED18 interactions. As shown in Fig. 6e , a clear YFP signal was detected in the nucleus when MED18-Yc and SUF4-Yn proteins were transiently co-expressed in N. benthamiana leaves demonstrating physical interaction. MED18-HA co-precipitated with Myc-SUF4 in co-IP experiments from N. benthamiana leaves confirming the BiFc data ( Supplementary Fig. 5c ). We further validated in vivo interaction in Arabidopsis transgenic plants where MED18-HA co-precipitated with Myc-SUF4 ( Fig. 6f ). Thus, multiple interaction data clearly indicate that MED18 physically interacts with SUF4 and likely suppresses its function in FLC transcription. SUF4 is a zinc finger-containing TF that is required for delayed flowering by promoting the FLC expression. SUF4 binds to a cis -element of the FLC promoter and acts as part of the transcriptional activator complex [35] . MED18 regulates different steps of transcription As described in the previous sections, MED18 associates with the promoter regions of PTR3, ABI5 and FLC genes and directly regulates their transcription, indicating that MED18 is involved in the initiation of transcription ( Fig. 4 ). However, it was unclear whether Arabidopsis Mediator is also involved in elongation and termination of transcription. Such a possibility was explored by using MED18 target genes— PTR3 , ABI5 and FLC . ChIP-qPCR of MED18-HA;med18 plants was used to study the recruitment of MED18 to the coding and terminator regions of MED18 target genes. The coding and terminator regions of the three target genes were significantly enriched for MED18-HA ( Fig. 4 ). The associations of MED18 with ABI5 coding and terminator regions were enhanced by ABA. Similarly, the coding and terminator regions of FLC were enriched with MED18-HA. B. cinerea infection resulted in the enhanced recruitment of MED18-HA to the PTR3 coding and terminator regions, although a significant level of MED18 already occupies these regions before pathogen infection, consistent with high basal expression of PTR3. Thus, our observations suggest that Arabidopsis MED18 is involved in the initiation, elongation and termination of transcription of target genes. The binding of MED18 to the initiation, elongation and termination sites of target genes does not preclude an epigenetic role for MED18. MED18 regulates RNA Pol II occupancy To arrive at a mechanistic understanding of how MED18 regulates gene expression, we analysed Pol II occupancy to different sites of target loci in wild-type and med18 mutant backgrounds using specific Pol II polyclonal antibodies (AntiRPB2 antibody ChIP Grade, ab10338, Abcam) ( Fig. 7 ). The Pol II occupancy of the TATA box, coding and terminator regions of PTR3 gene is significantly higher in the wild type than in the med18 mutant after inoculation with B. cinerea ( Fig. 7 ). Pol II occupancy on ABI5 was severely reduced in med18 mutant compared with the wild type. The data are consistent with the reduced expression of PTR3 and ABI5 in the med18 mutant. Unexpectedly, significantly reduced Pol II occupancy was also observed at the FLC locus despite its enhanced expression in the med18 mutant ( Fig. 7 ). The RNA Pol II occupancy of Arabidopsis Actin2, Actin7 and Ubquitin 10 (UBQ10), TATA box, coding and terminator regions were not affected by the med18 mutation ( Supplementary Fig. 9b ). Overall, the Pol II occupancy followed the pattern of MED18-HA association with PTR3 and ABI5. 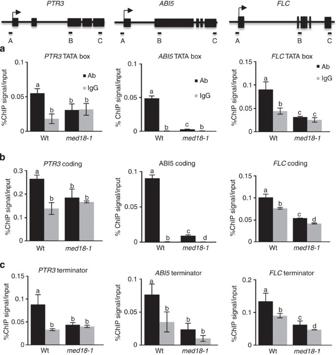Figure 7: MED18 regulates RNA Pol II occupancy of target genes. (a) ChIP analysis of RNA Pol II occupancy on TATA box, (b) coding and (c) terminator regions ofPTR3,ABI5andFLCgenes. ChIP analysis for RNA Pol II occupancy on individual genes regulated by MED18 was performed as described in the Methods section. The structures ofPTR3,ABI5andFLCgenes and positions of the primers used for qRT–PCR corresponding to the TATA box, coding and terminator regions are marked on the diagram at the top of the figure. ChIP was performed using RNA Pol II antibody. A control reaction was processed side-by-side with mouse IgG. ChIP- and input-DNA samples were quantified by real-time qPCR. The ChIP results are presented as percentage of input DNA. Error bars indicate s.e. (n=3). Figure 7: MED18 regulates RNA Pol II occupancy of target genes. ( a ) ChIP analysis of RNA Pol II occupancy on TATA box, ( b ) coding and ( c ) terminator regions of PTR3 , ABI5 and FLC genes. ChIP analysis for RNA Pol II occupancy on individual genes regulated by MED18 was performed as described in the Methods section. The structures of PTR3 , ABI5 and FLC genes and positions of the primers used for qRT–PCR corresponding to the TATA box, coding and terminator regions are marked on the diagram at the top of the figure. ChIP was performed using RNA Pol II antibody. A control reaction was processed side-by-side with mouse IgG. ChIP- and input-DNA samples were quantified by real-time qPCR. The ChIP results are presented as percentage of input DNA. Error bars indicate s.e. ( n =3). Full size image Impact of MED18 on H3 Lysine 36 tri-methylation Gene expression is the outcome of multiple mechanisms involving not only Mediator as a major transcriptional co-regulator but also post-translational histone modifications. We sought to determine the role of MED18 on histone H3 lysine methylation which is known to modulate gene expression in eukaryotes. ChIP using antibodies specific to H3 tri-methylations at lysine (K) residues 36 (H3K36me3) at chromatin of FLC, ABI5 and PTR3 loci were assessed ( Fig. 8 ). In med18 mutant, the H3K36me3 level on TATA box and coding regions of PTR3 and ABI5 genes were clearly reduced ( Fig. 8a,b ). The H3K36me3 on TATA box and coding regions of FLC were significantly enhanced relative to the wild-type plants ( Fig. 8c ). H3K36me3 is a mark of transcriptionally active chromatin [36] , [37] . The reduced H3K36me3 on PTR3 and ABI5 correlates with their reduced expression, while the enhanced H3K36me3 level on FLC is associated with its increased expression. The levels of H3K36me3 at the promoter and coding regions of the Actin2 gene used as a control here were not affected by the MED18 mutation confirming data from the previous sections on the specificity of MED18 functions ( Supplementary Fig. 9c ). The data suggest that MED18 may recruit different histone modification enzymes to regulate the levels of histone H3 methylation at the TATA box and coding regions of its target genes. 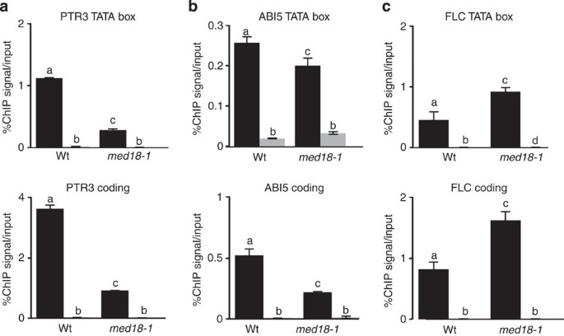Figure 8: MED18 modulates histone H3K36 tri-methylation at the coding region of target genes. (a) H3K36 tri-methylation at PTR3, (b) ABI5 and (c) FLC loci in wild-type andmed18mutant plants. ChIP was conducted with H3K36me3-specific antibodies (Abcam). ChIP for PTR3 was performed on 4-week-old plants at 2 dai withB. cinerea.AB15 ChIP was on 2-week-old seedlings treated with 50 μM ABA for 3 h. FLC ChIP was conducted on 2-week-old untreated seedlings. Data are representative of two independent experiments. Error bars indicate s.e. (n=3). Figure 8: MED18 modulates histone H3K36 tri-methylation at the coding region of target genes. ( a ) H3K36 tri-methylation at PTR3, ( b ) ABI5 and ( c ) FLC loci in wild-type and med18 mutant plants. ChIP was conducted with H3K36me3-specific antibodies (Abcam). ChIP for PTR3 was performed on 4-week-old plants at 2 dai with B. cinerea. AB15 ChIP was on 2-week-old seedlings treated with 50 μM ABA for 3 h. FLC ChIP was conducted on 2-week-old untreated seedlings. Data are representative of two independent experiments. Error bars indicate s.e. ( n =3). Full size image The molecular and biochemical mechanisms of how Mediator and its subunits govern expression of genes are still obscure particularly in plants where the functions of neither individual components nor the complex as a whole have been studied. The cellular and physiological functions of many Mediator subunits, including that of MED18, are unknown. In the current study, we demonstrate that MED18 plays significant roles in multiple biological functions, including plant responses to microbial infection, environmental signals regulating flowering and germination. At the cellular level, MED18 interacts with structurally distinct TFs to regulate target genes through which physiological responses are regulated. Interestingly, our studies also demonstrate that MED18 is recruited to different regulatory regions of target genes, including sites of transcriptional initiation, elongation and termination, suggesting contribution to the various stages of transcriptional control of gene expression. The association of MED18 with the terminator regions of target genes is consistent with the role of yeast Med18 in termination of transcription [38] . MED18 provides a bridging function between at least three different TFs, upstream signals and target genes producing positive or negative transcriptional outputs depending on its partner’s activator or repressor functions. This bridging function is further supported by the strong MED18 dependence of Pol II occupancy on target genes. The interactions between MED18, TFs and their target genes are summarized in the model for MED18 functions ( Fig. 9 , Supplementary Fig. 12 ). MED18 interacts with ABI4, YY1 and SUF4 TFs that are known to bind to different DNA sequences in their respective target genes performing different physiological functions. First, MED18 interaction at the ABI4-binding site of ABI5 modulates ABI5 gene expression, consistent with the positive role of MED18 on ABA responses. The impaired responses to ABA, reduced expression of ABI5 in med18 mutant and physical interaction with ABI4 demonstrate the critical role of MED18 in ABA responses. Interestingly, the disease resistance and ABA response functions of MED18 appear independent. Second, the negative regulation of GRX480, GRXS13 and TRX-h5 is clearly mediated by MED18 interaction with the transcriptional repressor YY1. YY1 maintains normal expression of GRX480, GRXS13 and TRX-h5 that are plant susceptibility factors to infection. Third, SUF4 interaction with MED18 plays a critical role for normal expression of the floral repressor FLC. However, the regulation of FLC is generally more intricate with other factors and regulatory processes involved. Mutation in SUF4 results in early flowering by reducing FLC gene expression [39] . The genetic data suggest that SUF4 and MED18 have contrasting functions. In the wild-type background MED18 may suppress the function of SUF4 in promoting FLC expression. Congruent with this, the med18 mutant exhibits enhanced FLC expression and extremely delayed flowering, which suggests the function of the wild-type MED18 protein is to promote flowering. This is consistent with our observation that MED18 suppresses SUF4 function through physical interaction and association at the FLC locus. Fourth, MED18 regulates PTR3 through direct association with the PTR3 regulatory regions. The intermediary TF through which this association occurs is not known. Together, the above data suggest that MED18 functional specificity and its role in activation or repression of gene expression are conferred by the sequence-specific DNA-binding zinc finger (YY1, SUF4) or ERF/AP2 (ABI4) domain TF proteins in response to upstream extra- and intracellular cues. Overall, MED18 is involved in multiple and seemingly independent biological functions and cellular processes. 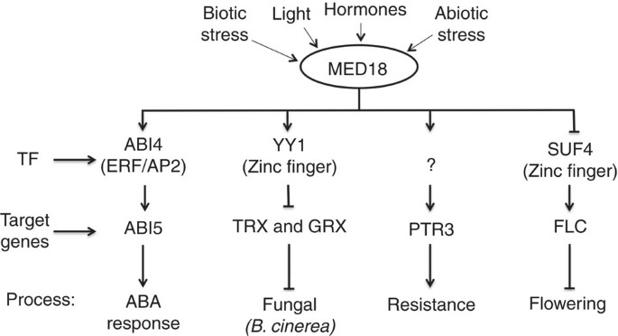Figure 9: Model showing the functions of MED18 and its partners. MED18 is required for signaling from upstream regulators to downstream components through interaction with transcription factors ABI4, YY1 and SUF4 to regulate plant responses to ABA, infection and flowering time, respectively. Those interactions directly regulate the expression of the corresponding target genesABI5,TRX-GRX,PTR3andFLCgenes. The transcription factor mediating PTR3 regulation by MED18 is unknown. Figure 9: Model showing the functions of MED18 and its partners. MED18 is required for signaling from upstream regulators to downstream components through interaction with transcription factors ABI4, YY1 and SUF4 to regulate plant responses to ABA, infection and flowering time, respectively. Those interactions directly regulate the expression of the corresponding target genes ABI5 , TRX-GRX , PTR3 and FLC genes. The transcription factor mediating PTR3 regulation by MED18 is unknown. Full size image Plant responses to infection involve specific and broad reprogramming of gene expression. MED18 is required to integrate and transmit defence-related signals from TFs to the transcriptional machinery contributing to the up and downregulation of diverse immune factors. Interestingly, markers of canonical immune response pathways such as effector-triggered immunity, particularly R -genes, PAMP-triggered immunity, systemic acquired resistance and JA/ET-mediated such as responses show no altered gene expression responses in med18 mutant. Thus, MED18 represents a novel immunity regulator that functions distinctly from other immune response factors. The immune response function of MED18 is carried out through at least two mechanisms involving activation (PTR3) and suppression (thioredoxins and glutaredoxin) of gene expression. PTR3 is a di- and tri-peptide transporter implicated in plant responses to wounding and infection [30] , [40] . It is possible that deficiency in the uptake of amino acids compromises the synthesis of some defence compounds. We identified Arabidopsis YY1 as a direct transcriptional repressor of TRX and GRX genes, connecting deregulation of redox homeostasis to impaired plant immunity. Our data also link Mediator function to redox homeostasis through interactions with YY1. Although the function of Arabidopsis YY1 is unknown, the metazoan YY1 is a multifunctional protein that activates, represses or initiates transcription of a diverse assortment of genes [41] . Both Arabidopsis yy1 and med18 mutants show deregulated and extremely high levels of GRX and TRX gene expression. Interestingly, other stress-related genes show normal expression in the mutant lines. Thus, MED18 and YY1 are not universal repressor of stress response gene expression but mediate transcriptional control of specific regulons. Some Arabidopsis GRX and TRX proteins are virulence targets for necrotrophic fungi [26] , [28] . GRXS13 facilitates infection by B. cinerea and the grxs13 mutant is resistant to the fungus [26] . TRX-h5 is required for victorin sensitivity mediated by LOV1 in Arabidopsis [42] and the trx-h5 mutant is insensitive to victorin. Interestingly, the victorin toxin from C. victoriae interacts with thioredoxin TRX-h5 (ref. 28) [28] . This interaction is recognized by the NBS-LRR R-protein LOV1 leading to sensitivity to the toxin and susceptibility to the pathogen [28] . TRX and GRX are key players in the cellular redox regulatory network whose perturbation by virulence factors from fungal necrotrophs may promote susceptibility. Alternatively, pathogen-activated GRX/TRX may modify other targets which then result in general activation of susceptibility mechanisms. Thus, their extreme deregulation in the med18 mutant may partly account for its enhanced susceptibility by altering the functions of multiple targets. Histone lysine 36 tri-methylation, often considered a mark of transcriptionally active chromatin, is clearly altered in the med18 mutant at target loci. Consistent with its reduced expression in med18 mutant, H3K36me3 was reduced at the PTR3 and ABI5 loci. However, the H3K36me3 level was enhanced at the FLC-TATA box and coding regions. Although MED18 clearly affects histone methylation, how this is accomplished is unclear and needs further studies. It is likely that MED18 interacts with histone methylation enzymes or other factors that co-recruit histone methylases. Because of the role of Mediator in global, specific, as well as basal and stress-induced gene expression, plants provide a robust genetic system to study Mediator functions and its role in plant adaptive responses to a changeable environment. Whether MED18 becomes a repressor or promoter of expression of its target genes is determined by its interacting partners. In conclusion, the genetic, molecular and RNA-seq analyses described here suggest that MED18 is a critical regulator of transcription with significant impact on plant responses to intra- and extracellular signals impacting diverse physiological and cellular processes. Plant materials Arabidopsis thaliana plants used in this study including the WT (Col-0) and mutants med18-1 (Sail_ 889_C08), med18-2 (SALK_027178C), ptr3-2 (SALK _003119C ), ptr3-3 (WiscDsLoxHs034_10D/Stock: CS903244), ying yang1-1 (SALK_071311C) , ying yang 1-2 (SALK_SALK_040806C) , abi4 and abi5 were obtained from Arabidopsis Biological Resource Center (ABRC) and confirmed by PCR to verify the mutant genotypes. Transgenic plants expressing MED18-HA and YY1-MYC were generated by agrobacterium-mediated transformation. The transgenic plants were selected on media containing hygromycin or the herbicide basta as selectable markers. MED19-HA and YY1-MYC transgenic plants expressing the respective proteins were selected on western blots using MYC or HA-specific antibodies, according to the manufacturer’s instructions. Plant growth conditions and diseases assays Arabidopsis plants used for disease assays were grown on soil in growth chamber with light intensity (140 to 150 μE m −2 s −1 ), temperature (24 °C), relative humidity (70%) and a 12 h light/12 h dark cycle. For seedling hormone response assays, seeds were plated on Murashige and Skoog (MS) medium at 22 °C with a 16 h light/8 h dark photoperiod with light intensity of 120 μE m −2 s −1 . Seeds for hormone assays were harvested at the same time. N. benthamiana plants for co-IP and BiFC analysis were grown at 22 °C with a 16 h light/8 h dark photoperiod with light intensity of 120 μE m −2 s −1 . B. cinerea, A. brassicicola and P. syringae disease assays were previously described [43] . Briefly, A. brassicicola strain MUCL20297 was grown on potato dextrose agar, and spores were suspended in distilled water for plant inoculation. A plant response to B. cinerea was tested by spraying on whole plants by spraying a spore suspension (2 × 10 5 spores per ml) in Sabouraud maltose broth buffer. The disease assay for A. brassicicola was performed on detached leaves. In both cases, inoculated plants were kept under a transparent cover to maintain high humidity. RNA extraction and gene expression analyses Total RNA was isolated with Trizol reagent according to the manufacturer’s instructions (Sigma). DNase treatment, complementary DNA synthesis and quantitative RT–PCR were performed according to the manufacturer’s instructions (New England BioLabs) using gene-specific primers ( Supplementary Table 1 ) with Arabidopsis Actin2 as an endogenous reference for normalization. RNA-seq analysis RNA sequence data were generated by Illumina sequencing platform according to Illumina protocols. Sequence quality was assessed with the FastQC (Version 0.10.0) program. Quality trimming was done with the FASTX toolkit (Version 0.0.13) with minimum quality score of 30 and minimum length of 50 nt. The quality trimmed reads were mapped against the Arabidopsis reference genome (TAIR10) with Bowtie2 (Version 2.0.0-beta6) and default parameters [44] . HTSeq (Version 0.5.3) was used to generate raw read counts from each sample for each gene feature using Bowtie2 generated mapping files and the Arabidopsis gene annotation file. Read counts for each sample were merged using custom in-house perl script and subsequently used for analysis of downstream differential gene expression. Differential expression (DE) analysis across different conditions between samples was carried out using ‘ R ’ (Version 2.15.1) and different methods of limma package [45] , [46] , [47] . Basic exploration of the read count data file, such as accessing data range, and library sizes was performed to ensure data quality. An edgeR object was created by combining the counts matrix, library sizes and experimental design using edgeR (v 2.6.1) package. Normalization factors were calculated for the counts matrix, followed by estimation of common dispersion of counts. Exact test for differences between the negative binomial distribution of counts for the two experimental conditions resulted in finding DE values, which were then adjusted for multiple hypothesis testing. Another method called as ‘voom’ from limma package (v 3.12.0) was also used for the DE analysis. The ‘voom’ function carries out log 2 transformation of counts followed by mean-variance estimation and assigning weight to each transformed value. Linear model coefficients are then calculated using limma’s design matrix, contrast matrix and log 2 -transformed values. The Linear model was fitted using the empirical Bayes method, and differences between counts for two experimental conditions were calculated, which was then adjusted for multiple hypothesis testing. Reads per kilobase of exon model per million mapped reads (RPKM) values were calculated for each sample using count data, followed by similar intermediate steps as described in the ‘voom’ method. Venn diagrams were generated displaying the DE genes with FDR <0.05 for comparisons between groups of samples using Venny ( http://bioinfogp.cnb.csic.es/tools/venny/index.html ). Biomolecular fluorescence complementation assays Vectors for Biomolecular Fluorescence Complementation (BiFC) (pFGC-N-YFP and pFGC-C-YFP) were previously described [48] . Full-length coding sequence of MED18 was inserted into pFGC-C-YFP and ABI4, YY1 or SUF4 coding sequence was inserted into pFGC-N-YFP. The plasmids were introduced into Agrobacterium tumefaciens (strain GV3101) and infiltrated into N. benthamiana leaves as described previously [49] . Forty-eight hours after infiltration, tissues were examined with a Zeiss LSM710 confocal microscope for interaction, and images were superimposed with Zeiss LSM710 software. Co-IP assays The full-length coding region of MED18 fused with the HA tag (MED18-HA) was cloned after the cauliflower mosaic virus 35S promoter into a modified version of binary vector pCAMBIA99-1. The full-length complementary DNA sequences of YY1, ABI4, and SUF4 were fused with the myc tag (Myc-YY1, Myc-ABI4 and Myc-SUF4) and cloned into binary vector pBA-Myc under 35S promoter. These constructs were transferred into A. tumefaciens strain GV3101. The combinations of MED18-HA and Myc-YY1, MED18-HA and Myc-ABI4, or MED18-HA and Myc-SUF4 were co-infiltrated into N. benthamiana . Thirty hours after infiltration, proteins were extracted in buffer (50 mM Tris-HCl, pH7.5, 100 mM NaCl; 2 mM EDTA; 1 mM NaF; 1 mM NaVO3; 1 mM PMSF; 10 mM β-glycero phosphate; 0.1% (v/v) Triton X-100; 0.5% (v/v) Nonidet P-40; and 1 × protease inhibitor cocktail). After cleaning by centrifugation at 12,000 g for 10 min, 1 ml of the supernatant was incubated with 10 μl of anti-HA-conjugated agarose beads (Sigma-Aldrich) for 12 h at 4 °C. The co-IP products were washed with the extraction buffer four times and then detected on a western blot. Similar co-IP procedures were used for co-IP from transgenic Arabidopsis plants that express epitope-tagged MED18-HA, Myc-YY1 or Myc-SUF4. In this case, the experiments were conducted on 2-week-old Arabidopsis seedlings. ChIP-qPCR ChIP was performed essentially as described [50] . For ABI4 target genes, 35S:MED18-HA; med18-1 transgenic seedlings were grown on MS medium for 3 weeks and treated with 50 μM ABA for 1 h. Chromatin was immunoprecipitated with HA antibody (Covance). ChIP-qPCR was performed with specific primers to the ABI4-binding regions and TATA box on the ABI5 promoter. A control ChIP with immunoglobulin G was run in parallel. For disease response genes, 4-week-old 35S:MED18-3xHA/ med18-1 transgenic plants were grown on soil in a growth chamber. Plants were inoculated with B. cinerea and diseased leaf sample collected at 36 h after inoculation and HA antibody was used to precipitate the protein–DNA complex. For flowering genes, 15-day-old seedlings grown on MS medium were sampled without any additional treatment. To determine DNA-directed RNA Pol II occupancy, wild-type and med18-1 mutant plants were treated similar to experiments in MED18-HA occupancy assays. Histone lysine methylation assays were conducted with specific antibodies according to the manufacturer’s (Millipore) instructions. All qRT–PCR primers are listed in Supplementary Table 1 . Accession codes: GenBank accession numbers for the genes used in this study are: YY1 ( NM_178992 ); MED18 (BT029378.1 GI: 117168218); SUF4 ( NM_102836.2 GI: 30692184); ABI5 ( NM_129185.3 ); ABI4 ( NM_129580.1 ); PTR3 ( NM_123973.3 GI: 30694875); FLC ( NM_001203343.1 GI: 334187572). The sequencing data have been deposited in the NCBI Sequence read archive under accession code SRP033777 . How to cite this article: Lai, Z. et al. MED18 interaction with distinct transcription factors regulates multiple plant functions. Nat. Commun. 5:3064 doi: 10.1038/ncomms4064 (2014).